Pesticide risk assessment in free-ranging bees is weather and landscape dependent The risk assessment of plant protection products on pollinators is currently based on the evaluation of lethal doses through repeatable lethal toxicity laboratory trials. Recent advances in honeybee toxicology have, however, raised interest on assessing sublethal effects in free-ranging individuals. Here, we show that the sublethal effects of a neonicotinoid pesticide are modified in magnitude by environmental interactions specific to the landscape and time of exposure events. Field sublethal assessment is therefore context dependent and should be addressed in a temporally and spatially explicit way, especially regarding weather and landscape physiognomy. We further develop an analytical Effective Dose (ED) framework to help disentangle context-induced from treatment-induced effects and thus to alleviate uncertainty in field studies. Although the ED framework involves trials at concentrations above the expected field exposure levels, it allows to explicitly delineating the climatic and landscape contexts that should be targeted for in-depth higher tier risk assessment. The current assessment of new plant protection products on bees requires a tiered sequence, the first tier covering lethal toxicity trials under controlled laboratory conditions, whereas higher tiers imply surveys under (semi-) field conditions. The laboratory trials are aimed at determining toxicity end points based on median Lethal Dose (LD 50 ) estimation following acute oral or contact exposure. LD 50 is designed to be a repeatable mortality parameter, returned by easily reproducible testing schemes. Conversely, there is currently a lack of standardized procedure, both at first and higher tiers, to quantify sublethal effects of pesticides, that is, behavioural impairments that may originate from non-lethal exposures. This assessment shortcoming was further underlined by recent studies on honeybees ( Apis mellifera ) and bumblebees ( Bombus terrestris ) carried out in free-ranging conditions [1] , [2] , [3] , [4] . Subsequently, the European governments have banned for 2 years, starting on December 2013, the use of three neonicotinoid pesticides as seed-coating treatment for some common flowering crops [5] , while calling for more studies in field-realistic conditions. A key issue currently uncovered by risk assessment schemes is whether the levels of pesticide residues found in nectar and pollen, and certified as sublethal in laboratory, can lead to adverse effects at the colony level on the field. To fill this gap, the European Food Safety Agency [6] has identified a need to set standards for the measurement of sublethal effects in free-ranging bees, for example, using homing experiments at home range scale [1] , [7] , [8] , although scaling up from individuals to colony remains a major conceptual and technical challenge [9] . Homing flight performance has been considered as a candidate criterion to reveal pesticide sublethal effects in free-ranging honeybees because it may provide useful information on a range of sublethal parameters [6] . Successful homing flight is contingent to the proper integration of multiple physiological and cognitive functions, including among others, orientation, spatial memory, associative learning, energetic metabolism and muscular flight activity. Therefore, homing experiments cover a wide spectrum of biological mechanisms of pesticides are liable to interfere with (ref. 6 ). For instance, neonicotinoids at sublethal concentrations alter the neurophysiological properties of Kenyon cells, which are the major neuronal components of the honeybee mushroom bodies where multisensory information signals are integrated [10] . This in turn will have detrimental effects on cognitive tasks such as memory retrieval and orientation, as revealed by increased Homing Failure (HF) [1] , [7] , [8] . Homing experiments are also relevant for field assessment because they are performed at the home range scale and because an increased probability of HF may be converted into a mortality parameter and implemented into exploratory models of colony population dynamics [1] , [11] , [12] . On the other hand, homing flights are conditioned by keystone environmental correlates of bee navigation, which are liable to interfere with the assessment of neonicotinoid sublethal effects in free-ranging conditions. Herein, Navigation Evironmental Correlate, thereafter abbreviated as NECs, refer to those extrinsic drivers of bee navigation and flight performances, comprising weather conditions (temperature, cloudiness or visibility of sun) and salient landmarks acting as visual cues for orientation [13] , [14] , [15] , [16] , [17] , [18] , [19] , [20] , [21] , [22] . Homing honeybees rely on a network of learned interconnected vectors for orientation [18] , conceptualized as memorized distances and directions among known locations. They further have the ability to derive novel shortcut vectors from the integration of two or more previously learned vector flights [19] . Honeybees retrieve the directional components of vector flights based on the sun as a celestial cue, but also on known landmarks whenever the sun compass or any spot of polarized light in the sky are masked by clouds [16] , [19] , [21] . Navigation in honeybees is further driven by temperature. Ambient temperature affects metabolism and flight speed [17] , for instance with lower wingbeat frequency and higher energy expenditure per wingbeat as ambient temperature decreases from 37 °C to 19 °C (ref. 22 ). Overall, temperature jointly with the availability of the sun compass and of the visual landmarks as orientation cues are regarded as key NECs. In this study, using HF as a paradigm for field assessment of pesticide risks to honeybees, we tested whether the neonicotinoid thiamethoxam interacts with NECs, potentially changing the latent sublethal effects among experimental contexts. First, we establish a generic dose–response function of HF, covering a broad range of sublethal exposure levels (non-exposed control bees and treatments from LD 50 /12 to LD 50 /2, with the LD 50 estimated at 5 ng per bee (ref. 23 )). Second, we test whether the specific weather, as well as landscape context at the time and place of individuals’ release, may modulate the expression of generic dose–response function through an interaction effect with thiamethoxam exposure. As the dose–response function proved to be highly context dependant, we finally propose analytical solutions to explicitly handle the resulting uncertainty. Following the LD principle, we computed the ED required for reaching a given sublethal effect size in free-ranging bees across a range of contexts. The ED framework is designed (i) to assess how the risk to honeybees do vary with weather and landscape contexts and (ii) to explicitly delineate the areas where the effect is expected to be strongest and therefore should be targeted for in-depth higher tier risk assessment. This approach will help disentangle environment-induced effects from treatment-induced effects in field surveys and thus will contribute to alleviate uncertainty in the assessment of pesticide side effects to bees. HF increases with oral exposure doses We carried out 60 homing trials (see Methods) involving 978 honeybee foragers from nine different colonies, released at 22 distinct locations 1 km away and monitored using RFID (Radio-Frequency IDentificationentification) microchips. The median probability of HF ranged from 0.17 in control trials to 0.40 in higher exposure (>0.5 ng per bee) trials. Controlling for the random effects of colonies and release points, the risk of HF, expressed as a 0-1 binary response variable, significantly increased with exposure dose in nanogram per bee (Linear Mixed Effect model (LME), n =978, Z=3.374, P <0.001), following the inverse logit function in equation 1. The dose–response function ( Fig. 1a ) returns a 46% increase of HF at a 1-ng dose (HF=0.259) compared with control (0.177). This effect size could be detected with a fairly high confidence level given our sample size ( a posteriori statistical power=99%, Fig. 1b ). Yet, a substantial variability was observed among trials, with high HF values in some control treatments, as well as low HF values at higher doses. Such high level of variability might be partly accounted for by NECs, as detailed below. 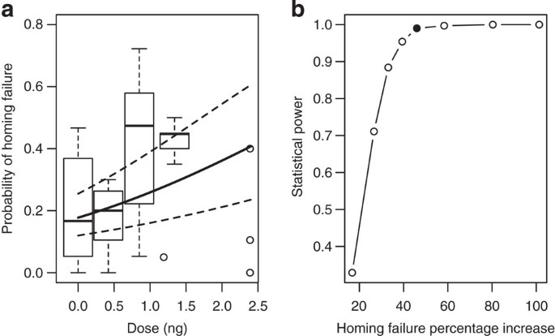Figure 1: Generic dose–response function of the risk of homing failure in exposed honeybees. (a) The predicted dose–response function (continuous line±estimate s.e. as dashed lines) derived from a binomial logit LME model, specifying random intercepts for colony and release point effects, withn=978 individuals split into 60 homing trials from 22 release points around nine colonies. Quartile boxes and dots overlaying predictions display observed homing failure proportions for trials with >15 individuals. (b) A posteriori statistical power analysis, appraising the ability of the LME to detect a significant homing failure dose–response with the current sample size. Statistical power was measured as the proportion of significant effects out of 1,000 simulated homing failure data sets randomly recomputed with a constrained effect size (percentage increase at 1 ng). The observed effect size (46% increase at 1 ng, filled dot) had a 99% chance of being detected given our sample size. Figure 1: Generic dose–response function of the risk of homing failure in exposed honeybees. ( a ) The predicted dose–response function (continuous line±estimate s.e. as dashed lines) derived from a binomial logit LME model, specifying random intercepts for colony and release point effects, with n =978 individuals split into 60 homing trials from 22 release points around nine colonies. Quartile boxes and dots overlaying predictions display observed homing failure proportions for trials with >15 individuals. ( b ) A posteriori statistical power analysis, appraising the ability of the LME to detect a significant homing failure dose–response with the current sample size. Statistical power was measured as the proportion of significant effects out of 1,000 simulated homing failure data sets randomly recomputed with a constrained effect size (percentage increase at 1 ng). The observed effect size (46% increase at 1 ng, filled dot) had a 99% chance of being detected given our sample size. Full size image The dose–response function is context dependent As predicted, NECs interacted significantly with the thiamethoxam exposure ( Table 1 , Fig. 2 ), therefore altering the shape and steepness of the generic dose–response function of HF ( Fig. 3 ). We focused our analyses on ambient temperature and availability of landmarks for orientation (total length of hedgerows and forest edges in the 1-km diameter area between the release point and the colony). Our measurements of solar radiations (W m −2 ), as an indication of sun compass availability, were strongly correlated with ambient temperature ( r s =0.68, P <0.001). When implemented into separate models, both temperature and solar radiations significantly influenced HF (LME; n =978, Z=−5.55, P <0.001 and n =978, Z=−4.58, P <0.001, respectively). But most importantly, they significantly interacted with thiamethoxam ( n =978, Z=−2.70, P =0.007 and n =978, Z=−2.55, P =0.010, respectively). However, temperature enabled a better fit to HF data than did solar radiations (Akaike Information Criterion (AIC) of LMEs with dose interactions=971.5 versus 983.6, respectively, with lower AIC indicating a better model fit), and was therefore considered as the most relevant weather-related NEC for investigating HF dose–response variations in our study. Table 1 Summary of the LME binomial models performed to assess the thiamethoxam dose-response function of honeybee homing failure and its interactions with NECs. 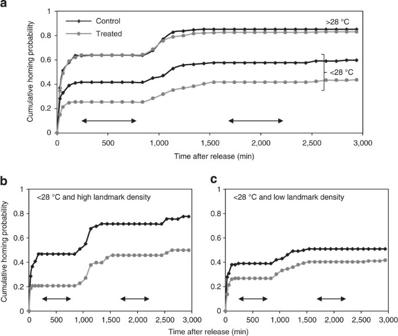Figure 2: Observed cumulative homing probability as a function of time lapse since honeybee release at 1 km from the colony. The interaction effects between treatment (control versus all doses confounded) and navigation environmental correlates (NECs) are depicted by successively splitting data based on (a) average temperature (28 °C) and (bandc) average landmark availability for orientation (4.2-km network of hedgerows and forest edges in the 1-km diameter area between the release point and the colony). Release time, that is, the origin of the temporal axis, was standardized among trials to 1630–1830 hours. Horizontal arrows indicate night time. Full size table Figure 2: Observed cumulative homing probability as a function of time lapse since honeybee release at 1 km from the colony. The interaction effects between treatment (control versus all doses confounded) and navigation environmental correlates (NECs) are depicted by successively splitting data based on ( a ) average temperature (28 °C) and ( b and c ) average landmark availability for orientation (4.2-km network of hedgerows and forest edges in the 1-km diameter area between the release point and the colony). Release time, that is, the origin of the temporal axis, was standardized among trials to 1630–1830 hours. Horizontal arrows indicate night time. 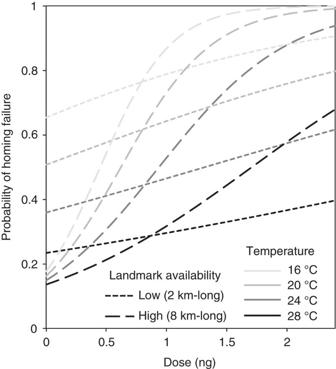Figure 3: Conditional predictions of the thiamethoxam dose–response function of honeybee homing failure probability. The predicted dose–response curves were computed for different combinations of temperature and landmarks availability, ranging from low landmark density (2 km long network of hedgerows and forest edges in the 1-km diameter area homing bees have to cover between the release point and the colony) to high landmark density (8 km). Intercepts show expected homing failure for non-treated bees in the context of the experiment. Intercepts therefore set the control value needed to calculate mortality rate due to homing failure,mHF, for honeybees exposed to a given dose. Full size image Figure 3: Conditional predictions of the thiamethoxam dose–response function of honeybee homing failure probability. The predicted dose–response curves were computed for different combinations of temperature and landmarks availability, ranging from low landmark density (2 km long network of hedgerows and forest edges in the 1-km diameter area homing bees have to cover between the release point and the colony) to high landmark density (8 km). Intercepts show expected homing failure for non-treated bees in the context of the experiment. Intercepts therefore set the control value needed to calculate mortality rate due to homing failure, m HF , for honeybees exposed to a given dose. Full size image The significant interactions ( Table 1 ) are merely depicted by the dissociated curves of homing statistics as a function of time after release ( Fig. 2 ). The Control - Treatment relative difference is negligible at higher temperatures and increases with decreasing temperature ( Fig. 2a ), as revealed by the negative Dose × Temperature interaction. At low temperatures ( Fig. 2b,c ), the homing gap between control and treated bees increases with landmarks availability. This is in accordance with the positive Dose × Landmarks interaction in model outputs ( Table 1 ). Notwithstanding, higher landmarks availability ( Fig. 2b ) was associated with overall lower HF than in more open landscapes ( Fig. 2c ). All in all, temperature appeared as the proximal driver of HF dose–response variations because it had steeper interaction estimates and with a greater relative importance than landmarks availability ( Table 1 ). However, landmarks availability was also an important environmental correlate of HF, judging from its pervasive occurrence in the set of best candidate models ( Table 2 ), and therefore should be explicitly accounted for whenever possible as well. In this study, none of the best candidate models of HF reached a predominant weight of evidence (all w i values <<90%, Table 2 ), indicating that it is advisable to resort to multimodel averaging to derive more conservative model predictions [24] . Table 2 Detailed set of all candidate explanatory LME models of homing failure in honeybees exposed to thiamethoxam, ranked by decreasing statistical support. Full size table The ED addresses context dependency Multimodel conditional predictions of the dose–response function ( Fig. 3 ) illustrate well the conclusion that NECs substantially modify the generic dose–response function of HF one may assess on the field. The dose–response curve is flattest at high temperatures in rather open landscapes (few landmarks available), and steepest at low temperatures in rather complex landscapes (high landmarks density). Those conditional dose–response functions ( Fig. 3 ) should be viewed as tentative predictions specific to our experimental context, and be further refined using additional data at the edges of temperature and landmark ranges. Homing experiments carried out with foragers familiar with the release point may also provide lower bound estimates of HF [1] . Because the spatial context, as revealed by landmarks density, is an important correlate of HF, one can derive spatially explicit maps of the expected HF for a given exposure level. However, given that consensus rarely emerges about field exposure levels [25] , one may instead map the exposure level required to reach a given effect size. A critical pesticide effect is reached when HF adds up to background mortality up to a point that entails a 35% reduction of colony size during an exposure event [6] , for example, during a 30-day oilseed rape flowering period. Using previously published colony dynamics parameters [11] , we found this critical slowdown is triggered at a mortality rate because of HF m HF >0.15, that is, if non-returning treated bees represent more than 15% of returning bees, one might expect from the control. For the sake of illustration, we therefore targeted a critical m HF value of 20% and mapped the corresponding required thiamethoxam dose, called ED 20 ( Fig. 4 ). All landscape units (pixels of the map) within the focus landscape (450-km 2 , Fig. 4 ) were assigned an ED 20 >0.320 ng per bee at 20 °C. This is greater than worst-case thiamethoxam residue intakes by foragers for 1 h flying (estimated to be <0.276 ng per bee for 20% sugar content nectar [26] ), meaning that the critical HF is unlikely to be reached over the focus landscape. 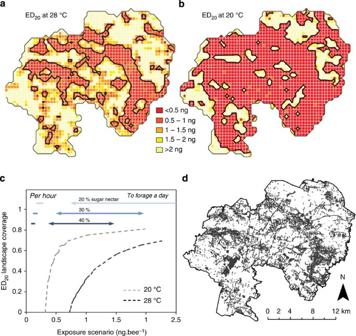Figure 4: Spatial assessment of the honeybee experimental homing failure, as delineated by the ED20(effective dose that leads to a 0.20 mortality rate due to homing failure). Mortality due to homing failure,mHF, is given by the relative difference of control versus treated homing probabilities. Conditional predictions show the sharp transition from (a) low-effect conditions at 28 °C to (b) high-effect conditions at 20 °C. Thick lines show the 1-ng ED20limits, delineating the landscape contexts where honeybees exposed to a 1-ng dose will be subject to a mortalitymHF>0.20. This area covers 34–75% of the whole landscape depending on the temperature (c), but may be much reduced if one focuses on lower exposure scenarios. Eventually, for doses <0.320 ng per bee at 20 °C, the landscape is expected to be exempt of critical homing failure risks (ED20landscape coverage=0%). For the sake of comparison, horizontal lines indicate worst-case scenarios of thiamethoxam intake by honeybees for 1 h flying, or to forage a day, based on 20–40% sugar nectars26. In particular, theper-hourexposure scenarios (for example, 0.184–0.276 ng per bee for a 20% oilseed rape nectar) fall in the 0% range for ED20landscape coverage. (d) ED20conditional predictions use the local geographic information on the network of hedgerows and forest edges. Figure 4: Spatial assessment of the honeybee experimental homing failure, as delineated by the ED 20 (effective dose that leads to a 0.20 mortality rate due to homing failure). Mortality due to homing failure, m HF , is given by the relative difference of control versus treated homing probabilities. Conditional predictions show the sharp transition from ( a ) low-effect conditions at 28 °C to ( b ) high-effect conditions at 20 °C. Thick lines show the 1-ng ED 20 limits, delineating the landscape contexts where honeybees exposed to a 1-ng dose will be subject to a mortality m HF >0.20. This area covers 34–75% of the whole landscape depending on the temperature ( c ), but may be much reduced if one focuses on lower exposure scenarios. Eventually, for doses <0.320 ng per bee at 20 °C, the landscape is expected to be exempt of critical homing failure risks (ED 20 landscape coverage=0%). For the sake of comparison, horizontal lines indicate worst-case scenarios of thiamethoxam intake by honeybees for 1 h flying, or to forage a day, based on 20–40% sugar nectars [26] . In particular, the per-hour exposure scenarios (for example, 0.184–0.276 ng per bee for a 20% oilseed rape nectar) fall in the 0% range for ED 20 landscape coverage. ( d ) ED 20 conditional predictions use the local geographic information on the network of hedgerows and forest edges. Full size image Our experiment demonstrates that HF in treated bees is highly context dependent, with temperature as a major proximal correlate of homing performance, and landmarks availability as a secondary, although interacting environmental correlate. Previous literature review [27] have already shown that some pesticides (pyrethroids) have greater toxicity at low temperatures (for example, below 28–30 °C), which could be related with impairments of neural mechanisms of thermogenesis rather than with troubles of flight muscular coordination or metabolic rate. Neonicotinoids may, however, involve different toxicological pathways. In particular, we cannot exclude that neonicotinoids interfere with the honeybee orientation system. Interestingly, the greatest treatment effect was measured during poor weather conditions in environments with a greater density of landmarks ( Fig. 2b ), suggesting that treated foragers had greater difficulties to recover and integrate the information on vector flights among learned landmarks and/or to derive novel shortcut vector flights [18] , [19] . This also matches the recent evidence from harmonic radar tracking surveys that honeybees experience difficulties in their homing flight pattern after non-lethal exposure to neonicotinoid pesticides [28] . When forced to split their route flight back to the hive into a vector phase based on sun compass and a homing search phase from a known landmark, exposed honeybees were less efficient in completing the second phase, which involves retrieval of remote memory [28] . This conforms well to our observation that higher landmark availability is associated with lower ED levels to reach the critical 20% HF ( Fig. 4 ). The spatially explicit predictions of ED 20 delineate consistent high-effect areas at medium temperatures ( Fig. 4a ). As temperature decreases, the high-effect area expands over most of the landscape, restricting low-risk areas to a few remote spots ( Fig. 4b ). However, further research is necessary to determine whether those low-effect refuges may be viewed as effect free for apiaries, or not. Indeed, those areas correspond to the most open landscapes ( Fig. 4d ) where both control and treated HF are high ( Fig. 2c ). They may thus rather be viewed as environments with greater challenge imposed upon honeybee navigation during poor weather conditions, where any treatment effect will be harder to detect. Notwithstanding, with the help of experts’ assessment of the field exposure levels [29] , [30] and how they compare with ED 20 values, this approach allows determining the proportion of the landscape at risk of detrimental HF in case of exposure. We found the worst-case daily cumulative thiamethoxam residue intake (for example, 0.736–2.944 ng per bee for 20% sugar content nectar [26] ) entails a 70–80% landscape ED 20 coverage ( Fig. 4c ). However, the residue intake cumulated over an entire foraging day is not perceived as a valid, field realistic, exposure scenario for free-ranging bees, particularly in the case of transient behavioural observations such as homing tests [6] , [26] . Alternatively, one should focus on an hourly basis, best suited for studying behavioural issues at the scale of foraging bouts. Here, the worst-case scenarios of residue intakes by foragers for 1 h flying (estimated to be <0.276 ng per bee for 20% sugar content nectar [26] ) are unlikely to reach critical ED 20 levels at 20 °C in any landscape unit of the focus area (all ED 20 >0.320 ng, Fig. 4c ). However, given the rather narrow gap between those two end points, it might be critical to refine estimations of field dietary residue intakes and associated uncertainty levels, as well as the occurrence likelihood of worst-case scenarios in field conditions. In conclusion, the assessment of sublethal effects in free-ranging honeybees may be highly context dependent. The strong context dependency helps understand the difficulty to establish consistent links between laboratory-based toxicological assays and field observations [29] , [31] . This compromises the applicability of HF as a paradigmatic approach to the sublethal risk assessment in field conditions because neonicotinoids will not return repeatable, generic, dose–response functions. Instead, we argue that field assessment schemes should either (i) provide details about landscape and weather conditions, (ii) use thoroughly standardized landscape and weather conditions or (iii) cover an extensive range of contexts along with substantial sample sizes. In addition, large-scale epidemiological surveys aimed at exploring potential links between colony losses and phytosanitary practices across regions or countries should whenever possible incorporate interacting climate or landscape covariates. In that respect, the ED framework, although involving trials at a range of concentrations above the expected field exposure levels, has the potential to become an operative tool to help toxicologists identify some specific contexts that should deserve particular attention in the course of higher tier risk assessment. Homing experiments This homing study covers ongoing experiments from springs 2011 (Experiment 2 in Henry et al. [1] ) and 2012, using RFID individual monitoring [32] coupled with landscape-scale characterization of salient landmarks as orientation cues [33] . We analysed the homing statistics of 978 individual honeybees obtained from nine colonies in the course of 60 distinct homing trials. A homing trial was defined as a group of about 15–20 bees (mean and s.d.=16.3±2.9) released at one given site after receiving an acute oral thiamethoxam or control treatment ( Table 3 ). Five thiamethoxam doses were chosen so as to cover a broad range of LD 50 fractions (from LD 50 /20 to LD 50 /2, with LD 50 =5 ng per bee) and to increase the ability of the study to delineate a consistent dose–response function. Real experimental doses were subsequently titrated at 0.42–2.39 ng per bee (LD50/12 to LD50/2). This range lies above the worst-case thiamethoxam residue intakes by foragers expected for an hour flying (for example, 0.184–0.276 ng per bee with an average 20% sugar content nectar of treated oilseed rape [26] ). However, this did not compromise the study, which was first and foremost designed to establish a dose–response profile and its context dependency. The dose was administered to bees in 20 μl of a 50% sucrose solution. Bees were kept for a 40-min assimilation period before release. Their homing flight was monitored by RFID microships glued on their thorax and a series of ad-hoc readers placed at the colony entrance [1] , [32] . Table 3 Sample size allocation among trials, colonies and experimental doses. Full size table Field experimental design A. mellifera ligustica strain colonies were headed by sister queens bred the previous summer during the same grafting session and wintered in nuclei, then set up on experimental location in April. Colonies were disposed >3 km apart from each other (nearest distance range=3.7–10.4 km, Fig. 5 ), across the ECOBEE platform, western France [34] . Homing experiments were performed after oilseed rape flowering period to avoid interferences with field treatments. Twenty-two release sites, located 1 km away from colonies (two to six per colony, Fig. 5 ) were chosen so as to maximize the overall variability of their landmark density values (total length of hedgerows and forest edges included in the 1 km diameter circular area homing bees need to cross over to get back to their colony). Treated and control groups were released simultaneously at each trial, and at a standardized time among trials (16:30–18:30 h). 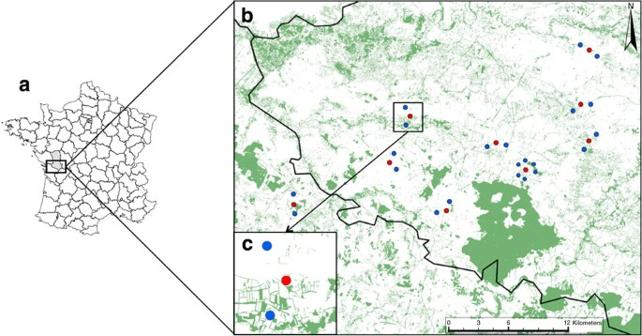Figure 5: Map of the study area and location of experimental colonies. (a) Location of the study area in western France. (b) Location of the experimental colonies (red) and associated release points (blue) superimposed on the woody vegetation layer (Institut Géographique National) illustrating regional variations in landscape complexity. The solid black line delineate regional boundaries. (c) Details of one experimental site, emphasizing the contrasted landscape context between release points. Figure 5: Map of the study area and location of experimental colonies. ( a ) Location of the study area in western France. ( b ) Location of the experimental colonies (red) and associated release points (blue) superimposed on the woody vegetation layer (Institut Géographique National) illustrating regional variations in landscape complexity. The solid black line delineate regional boundaries. ( c ) Details of one experimental site, emphasizing the contrasted landscape context between release points. Full size image NECs Experiments were exclusively carried out under weather compatible with current foraging activity, that is, excluding rainy, cold (<15 °C) and windy (>15 km h −1 ) conditions [35] . Ambient temperature was measured at the point and time of release. Solar radiations (W m −2 , averaged hourly) were measured using a pyrometer placed in the centre of the study area, as an indication of cloudiness, and recorded on a continuous basis. Landmarks availability was measured as the total length (km) of hedgerows and forest edges ( sensu [33] ) in the 1-km diameter area homing bees have to cover between the release point and the colony. Data analysis HF was defined as an absence of RFID record during the 7 days post-release, and was coded as a 0/1 binary response variable (return/no return, respectively). In a first step, the binary data were analysed in relation with exposure doses using a LME to establish a generic dose–response function. To conform the assumption of independent outcomes in the binary homing observations, the identity of experimental colonies and of release points were included as random grouping variables, along with the dose effect as fixed explanatory variable. A statistical power analysis was performed a posteriori to assess the ability of the LME to detect a significant HF dose–response with the current sample size. Statistical power was measured as the proportion of significant effects out of 1,000 simulated HF data sets recomputed from random binomial distributions with probability constrained on a range of potential effect sizes. In a second step, NECs were added to the LME model as additional correlates of HF, interacting with the dose effect. All the possible two- and three-way interactions among explanatory variables were considered within the frame of a multimodel inference procedure [24] . The most plausible combinations of explanatory variables were determined using the AIC of model parsimony, considering model fit and complexity. We used a ΔAIC<2 cutoff rule to define the most parsimonious models and determine the relative importance and significance of candidate exploratory variables. Variables were centered to mean=0 and standardized to s.d.=0.5 before the analysis, so that their respective effects are given in s.d. units and therefore are readily interpretable in terms of effect size and comparable among each others. How to cite this article: Henry, M. et al. Pesticide risk assessment in free-ranging bees is weather and landscape dependent. Nat. Commun. 5:4359 doi: 10.1038/ncomms5359 (2014).